Adaptive rewiring aggravates the effects of species loss in ecosystems Loss of one species in an ecosystem can trigger extinctions of other dependent species. For instance, specialist predators will go extinct following the loss of their only prey unless they can change their diet. It has therefore been suggested that an ability of consumers to rewire to novel prey should mitigate the consequences of species loss by reducing the risk of cascading extinction. Using a new modelling approach on natural and computer-generated food webs we find that, on the contrary, rewiring often aggravates the effects of species loss. This is because rewiring can lead to overexploitation of resources, which eventually causes extinction cascades. Such a scenario is particularly likely if prey species cannot escape predation when rare and if predators are efficient in exploiting novel prey. Indeed, rewiring is a two-edged sword; it might be advantageous for individual predators in the short term, yet harmful for long-term system persistence. The initial failure of one component (node) in a complex network can potentially lead to cascading failures of other components with disastrous effects on the network [1] , [2] . For instance, in ecological networks loss or declining abundance of one species can trigger extinctions of other dependent species [3] , [4] , [5] , [6] , [7] , in the worst case leading to a complete system collapse [8] . Both top-down driven [9] and bottom-up driven secondary extinctions [5] have been documented in ecological communities. Looking at bottom-up driven secondary extinctions, the loss of a plant species might cause extinctions of herbivores specializing on that particular plant [5] , [10] , [11] . Likewise, specialized parasites might go secondarily extinct following the loss of their host species [5] . The possible frequency and extent of such secondary extinctions as well as mechanisms that might prevent them is attracting considerable current interest (for recent reviews see refs 12 , 13 ). Two possible mechanisms that may buffer against bottom-up driven secondary extinctions in ecological networks are the forming of new feeding links (rewiring) and compensatory readjustment of flows through remaining links ( Fig. 1 ). In food webs (or plant-pollinator networks) a predator (pollinator) species might switch to a new prey (plant) species following the extinction of its original prey (plant) species [11] . It has been suggested that such rewiring, as well as other adaptive trophic behaviour, should promote network persistence [14] and decrease the risk of cascading extinctions [11] , [15] , [16] , [17] , [18] , [19] . However, in antagonistic networks like food webs and parasite-host networks, rewiring and reallocation of feeding efforts following prey (host) species loss could lead to increased predation pressure (parasite load) on the remaining prey (host) species in the network. High grazing (predation) pressure have been found to reduce diversity of resource species in natural ecosystems [20] , [21] and to increase extinction risk of primary producers in model food webs [22] . It is also well-known that high densities of herbivores released from predation can result in destructive overgrazing of primary producers in both terrestrial and aquatic ecosystems [9] , [23] . Together these observations points to potential negative consequences of rewiring. Indeed, effects of predator diet shifts observed in some natural ecosystems [24] , [25] and inferred from the fossil record [26] indicate that rewiring might actually trigger rather than prevent extinction cascades. Thus, instead of decreasing the risk of network collapse, adaptive rewiring could increase it. 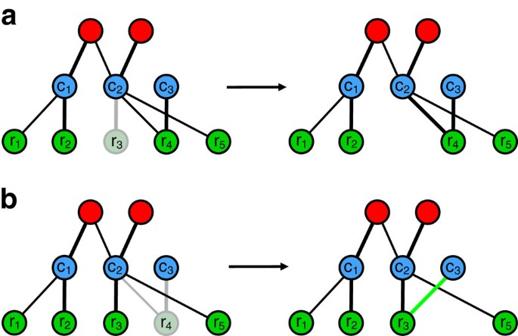Figure 1: The response of adaptive consumers to resource species loss. (a) Redistribution of feeding efforts and (b) rewiring. (a) Consumer c2loses its preferred resource r3and redistributes its feeding efforts by selecting another of its original resources, r4, as the preferred one. (b) Consumer c3loses its only resource and rewires (green link) to a new resource, r3. The new resource is randomly assigned from the set of resources belonging to the consumer which has the most similar set of prey (here consumer c2) as that of the rewiring consumer itself (here consumer c3). Consumer similarity,J, with respect to their sets of prey,R(c1)={r1, r2},R(c2)={r3, r4, r5} andR(c3)={r4}, is quantified using the Jaccard index of similarity;J(c3, c2)=(|c3∩c2|) / (|c3∪c2|)=0.33 andJ(c3, c1)=(|c3∩c1|) / (|c3∪c1|)=0. Top consumers (red), intermediate consumers (blue) and primary producers (green). Thick links indicate preferred resources. Figure 1: The response of adaptive consumers to resource species loss. ( a ) Redistribution of feeding efforts and ( b ) rewiring. ( a ) Consumer c 2 loses its preferred resource r 3 and redistributes its feeding efforts by selecting another of its original resources, r 4 , as the preferred one. ( b ) Consumer c 3 loses its only resource and rewires (green link) to a new resource, r 3 . The new resource is randomly assigned from the set of resources belonging to the consumer which has the most similar set of prey (here consumer c 2 ) as that of the rewiring consumer itself (here consumer c 3 ). Consumer similarity, J , with respect to their sets of prey, R (c 1 )={r 1 , r 2 }, R (c 2 )={r 3 , r 4 , r 5 } and R (c 3 )={r 4 }, is quantified using the Jaccard index of similarity; J (c 3 , c 2 )=(|c 3 ∩c 2 |) / (|c 3 ∪ c 2 |)=0.33 and J (c 3 , c 1 )=(|c 3 ∩c 1 |) / (|c 3 ∪ c 1 |)=0. Top consumers (red), intermediate consumers (blue) and primary producers (green). Thick links indicate preferred resources. Full size image Earlier studies on rewiring in ecological networks are mainly based on a static (topological) approach that do not consider population dynamics (for example, refs 15 , 17 , 27 ). Such an approach precludes an exploration of the effects of top-down processes and hence the potentially negative effects of rewiring. Here we use a dynamical modelling approach—allowing positive as well as potentially negative effects of rewiring to be captured—to investigate how extinction-induced rewiring affects the persistence (proportion of species surviving for a given period of time) of food webs in a variable environment. Thus, we consider the effects of species population dynamics as well as environmental variability on the response of food webs to species loss and subsequent rewiring. We also indirectly account for demographic stochastic variation and other processes that affect small populations disproportionately by defining quasi-extinction thresholds. Such processes are likely to make resource species more vulnerable to extinction when suppressed to low levels by increased predation pressure from rewiring consumers. Using this modelling framework we investigate (i) the effects of rewiring on network persistence and how these effects are modulated by (ii) a rewiring cost (meaning that a consumer is less effective in exploiting novel resources), (iii) consumers’ feeding specialization and functional response and (iv) network structure. We analyse a broad spectrum of networks; four natural food webs—from marine, freshwater and terrestrial habitats—and three different types of computer-generated food webs—pyramidal, bipartite and probabilistic niche model webs. Our study shows that adaptive consumer rewiring induced by prey species loss increases rather than decreases the risk of cascading extinctions in food webs. This negative effect of rewiring is due to overexploitation of resources, which is particularly likely when predators are efficient in exploiting rare and novel prey. To conclude, forming of new feeding links by consumers adapting to the loss of prey does not rescue food webs from cascading extinction. These results have possible bearings on human exploitation of natural populations where large-scale rewiring has been documented [28] , [29] , [30] . Effects of rewiring on network persistence Generally, we find almost no positive effects of rewiring on food web persistence. 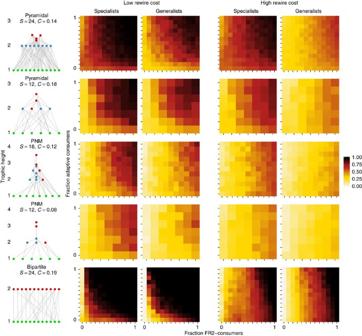Figure 2: Rewiring increases risk of cascading extinction—theoretical food webs. The proportion of species going extinct in pyramidal, PNM and bipartite food webs as a function of the fraction of adaptive consumers (FAdap) and the fraction of consumers with a type II (FFR2) and type III (1-FFR2) functional response. Dark colour indicates high proportion extinct species. Column 1 shows example topologies of all theoretical food web types. Column 2–3 and column 4–5 denote low and high rewire cost, respectively. Specialist consumers (strong preference for one prey) are shown in column 2 and 4, and generalist consumers (equal preference for each prey) are shown in column 3 and 5.Sdenotes number of species andCdenotes connectance. Green, blue and red nodes represent basal, intermediate and top species, respectively. The degree of correlation in the response of species to environmental variation,ρ, equals 0.75. Results are based on 50 replicate food webs for each scenario (each cell). On the contrary, the effect of rewiring on the persistence of both natural and computer-generated food webs ( Supplementary Table 1 ) is predominantly negative; the proportion of species going extinct increases with an increasing fraction of adaptive consumers in the webs ( Figs 2 and 3 and Supplementary Table 2 ). 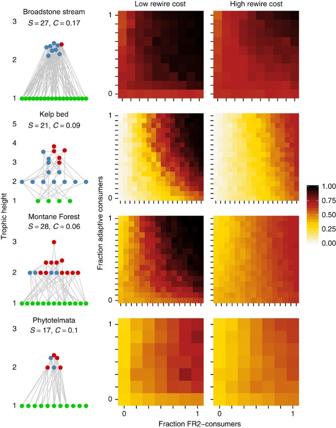Figure 3: Rewiring increases risk of cascading extinction—natural food webs. The proportion of species going extinct in natural food webs as a function of the fraction of adaptive consumers (FAdap) and the fraction of consumers with a type II (FFR2) and type III (1-FFR2) functional response. Dark colour indicates high proportion extinct species. Consumers have strong preference for one of their prey species (specialists). Column 1 shows the topologies of the natural webs. Column 2 and column 3 denote low and high rewire cost, respectively.Sdenotes number of species andCdenotes connectance. Green, blue and red nodes represent basal, intermediate and top species, respectively. The degree of correlation in the response of species to environmental variation,ρ, equals 0.75. Results are based on 50 replicate food webs for each scenario (each cell). For a subset of the food webs an expanded analysis using Latin hypercube sampling (LHS) of a larger parameter space is performed ( Supplementary Table 3 ). This expanded analysis also shows a very clear negative effect of rewiring on persistence, demonstrating the generality of the results ( Supplementary Fig. 1 ). The increased risk of extinction, caused by rewiring, affects species at all trophic levels ( Supplementary Fig. 2 and Supplementary Table 2 ). Furthermore, the negative effect of rewiring on long-term network persistence is present whether the consumers show strong preference for one prey species (specialist consumers) or equal preference for each prey species (generalist consumers), but is particularly pronounced when consumers are specialist. Overall, species are less likely to go extinct in food webs with generalist consumers than in webs with specialist consumers ( Fig. 2 , Supplementary Fig. 2 and Supplementary Table 2 ). In addition, the effect of rewiring is negative both when the correlation among species in their response to environmental variation is high ( Figs 2 and 3 ) and when it is low ( Supplementary Fig. 3 and 4 ). Overall, extinction risks are higher when correlation among species is low. Figure 2: Rewiring increases risk of cascading extinction—theoretical food webs. The proportion of species going extinct in pyramidal, PNM and bipartite food webs as a function of the fraction of adaptive consumers ( F Adap ) and the fraction of consumers with a type II ( F FR2 ) and type III (1- F FR2 ) functional response. Dark colour indicates high proportion extinct species. Column 1 shows example topologies of all theoretical food web types. Column 2–3 and column 4–5 denote low and high rewire cost, respectively. Specialist consumers (strong preference for one prey) are shown in column 2 and 4, and generalist consumers (equal preference for each prey) are shown in column 3 and 5. S denotes number of species and C denotes connectance. Green, blue and red nodes represent basal, intermediate and top species, respectively. The degree of correlation in the response of species to environmental variation, ρ , equals 0.75. Results are based on 50 replicate food webs for each scenario (each cell). Full size image Figure 3: Rewiring increases risk of cascading extinction—natural food webs. The proportion of species going extinct in natural food webs as a function of the fraction of adaptive consumers ( F Adap ) and the fraction of consumers with a type II ( F FR2 ) and type III (1- F FR2 ) functional response. Dark colour indicates high proportion extinct species. Consumers have strong preference for one of their prey species (specialists). Column 1 shows the topologies of the natural webs. Column 2 and column 3 denote low and high rewire cost, respectively. S denotes number of species and C denotes connectance. Green, blue and red nodes represent basal, intermediate and top species, respectively. The degree of correlation in the response of species to environmental variation, ρ , equals 0.75. Results are based on 50 replicate food webs for each scenario (each cell). Full size image Influence of rewiring cost and functional response The negative effects of rewiring on network persistence are particularly strong when the cost of rewiring is low, that is, when the predator is effective in exploiting its new prey species ( Figs 2 and 3 , Supplementary Figs 1–4 ). If the cost is high, the risk of overexploiting the new prey species, and thereby initiating an extinction cascade, is reduced. On the other hand, the higher the rewiring cost the less likely that the consumer will be able to survive on its new prey ( Fig. 4 ). Thus, if the rewiring cost is high the consumer is less likely to persist, whereas if the cost is low the risk that the rewiring consumer will trigger an extinction cascade is high. 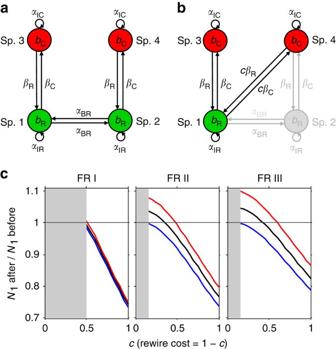Figure 4: Consequences of rewiring in a four species food web module. (a) Pre-extinction module; two consumers (red) feeding on one resource (green) each. (b) The module after extinction of one of the resources (species 2, grey). The extinction causes consumer species 4 to rewire to the remaining resource (species 1). (c) The ratio of the surviving resource’s equilibrium density after and before rewiring as a function of the cost of rewiring, 1−c. Panels show the ratio for functional response type I (analytically solved) and for functional response type II and III (numerically solved). The coloured curves represents different strengths of interspecific competition between resource species,αBR; blue curve (αBR=0), black curve (αBR=0.5) and red curve (αBR=1). Unfeasible (not all species have positive densities) part of the parameter range is shaded. Where systems are unfeasible, the rewiring consumer (species 4) has gone extinct following the extinction of its resource. (See also influence of rewiring cost and functional response in Results section.). Figure 4: Consequences of rewiring in a four species food web module. ( a ) Pre-extinction module; two consumers (red) feeding on one resource (green) each. ( b ) The module after extinction of one of the resources (species 2, grey). The extinction causes consumer species 4 to rewire to the remaining resource (species 1). ( c ) The ratio of the surviving resource’s equilibrium density after and before rewiring as a function of the cost of rewiring, 1− c . Panels show the ratio for functional response type I (analytically solved) and for functional response type II and III (numerically solved). The coloured curves represents different strengths of interspecific competition between resource species, α BR ; blue curve ( α BR =0), black curve ( α BR =0.5) and red curve ( α BR =1). Unfeasible (not all species have positive densities) part of the parameter range is shaded. Where systems are unfeasible, the rewiring consumer (species 4) has gone extinct following the extinction of its resource. (See also influence of rewiring cost and functional response in Results section.). Full size image Furthermore, the larger the proportion of consumers having a hyperbolic type II functional response, the more negative the effects of rewiring, that is, the higher the risk of species extinction and system collapse ( Figs 2 and 3 ). Only when almost all consumer species have a sigmoidal type III functional response is there a tendency for rewiring to lead to decreased extinction risks, especially for the top consumers ( Supplementary Table 2 ). Then consumers are less efficient in exploiting prey when prey densities are low ( Supplementary Fig. 5 ) and resource species will therefore be ‘protected’ from overexploitation (like in the case of adaptive diet choice of consumers which leads to decreased predation pressure on a prey species as its density decreases relative to other prey species [14] ). As a result, the negative effect of rewiring on the survival of primary producers will be less severe ( Supplementary Fig. 2 and Supplementary Table 2 ) and the risk of bottom-up extinction cascades thus decreases. The strong negative effects of rewiring in the scenarios where rewire costs are low and consumers have hyperbolic (type II) functional responses are corroborated by analytical work on a 4-species module ( Fig. 4 ). Consider a food web module with two consumer species and two competing resource species. Consumer species 3 feed on resource 1 and consumer species 4 feed on resource species 2 ( Fig. 4a ). Now, assume that resource species 2 goes extinct and consumer species 4 rewires to the remaining resource species 1. Then resource species 1 will be used by both consumer species ( Fig. 4b ). In the case of a linear functional response the population dynamics of the initial system can be described by the following system of differential equations: Here N i is the population density of species i , b R and b C are the intrinsic growth and mortality rates, respectively, α IR and α IC the strength of intraspecific competition in the resources and consumers, respectively, and α BR is the strength of interspecific competition between resource species. Finally, β C defines the per capita effect of a consumer on the growth rate of a resource and β R defines the per capita effect of a resource on the mortality rate of a consumer. Following extinction and rewiring the dynamics is given by the following system of differential equations: Here the parameter c , which takes values between 0 and 1, is introduced to explore the effects of a cost when the consumer that lost its original resource rewires to a novel resource. A low c means a high cost whereas a high c means a low cost. A high cost (low c ) means that the rewiring consumer species is poorly adapted to its new resource. Now, setting α IR and b R equal to unity, the equilibrium density of resource species 1 before ( ) and after ( ) the extinction of species 2 and the subsequent rewiring equals Now, if rewiring will have caused the density of resource species 1 to become closer to the quasi-extinction threshold and hence be exposed to a higher risk of extinction in a stochastically varying environment [31] . It can be seen that the fulfilment of the inequality is less likely when c is small (rewire cost is high), α BR is large (interspecific competition between resource species is strong) and α IC is large (intraspecific competition in consumer species is strong) ( Fig. 4c ). This is also the case when the functional response is of type II or III ( Fig. 4c ). Influence of network topology and type To investigate possible influences of network topology on the effects of rewiring on network persistence we perform a regression tree analysis ( Supplementary Figs 6–8 ) (the topological properties included in the analysis are described in Supplementary Tables 4 and 5 ). Only for pyramidal webs do we find some effects; 1) when consumers have strong preference for one prey species (specialists) and rewiring cost is high, impact of rewiring on network persistence is affected by connectance and 2) when consumers have equal preference for each of their prey (generalists) and rewiring cost is low, impact of rewiring is affected by connectance and average weighted prey vulnerability. Overall, topological properties have small effects on network persistence compared with other variables (rewire cost, type of functional response and prey preference distribution). However, there is a tendency for extinction risk to increase with increasing species richness ( Fig. 2 ). The most likely explanation for this is a negative relationship between species richness and average population density of species, meaning that populations are closer to the extinction threshold in species-rich networks than in species-poor ones ( Supplementary Fig. 9 ). In a variable environment, this will inevitably lead to an increased extinction risk [31] . Our analysis also shows that food web persistence decreases (extinction risk of species increases) with species richness both in the presence and absence of network rewiring. Thus, rewiring does not shift the relationship between species richness and persistence from a negative to a positive one (see also ref. 32 ). The effect of rewiring varies somewhat with network type, being more consistently negative for pyramidal and bipartite webs than for probabilistic niche model (PNM) webs. In PNM webs there is no clear negative effect of rewiring on network persistence when the cost of rewiring is high. A possible explanation for the less consistent effects of rewiring in the PNM webs is that the densities of basal species are, on average, higher in these webs than in the other web types, decreasing the risk of extinction ( Supplementary Fig. 9 ). Pattern of extinction We find that, on average, primary producers are the first to go extinct followed by consumer species. In the majority of cases primary consumers go extinct earlier than secondary consumers ( Supplementary Fig. 10 ). An example illustrating the path towards network collapse, for a scenario where all consumers are specialists and adaptive, have a type II functional response and where there is no cost of rewiring, is shown in Fig. 5 . In this very fragile worst case scenario, rewiring following an initial stochastic extinction of a primary producer triggers an extinction cascade: the initial extinction causes consumers to redistribute feeding efforts and rewire, which in turn causes extinction of a new prey species, and for each prey species that goes extinct the load on the remaining prey species becomes larger and larger until the whole network finally collapses. The same principle mechanisms are also at play in less extreme scenarios, though the consequences are less severe. The conclusion that rewiring leads to increased load on remaining prey species is corroborated by analytical work on a 4-species module ( Fig. 4 ); increased predation pressure following the extinction of one prey species and accompanying rewiring leads to reduced population size of the remaining prey. 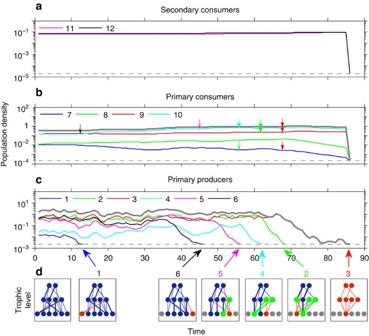Figure 5: Network collapse driven by resource species extinctions and consumer rewiring. Time series showing population dynamics for (a) secondary consumers, (b) primary consumers and (c) primary producers. Horizontal dashed lines: extinction thresholds. Thick grey lines: combined densities of (c) all primary producers and (b) all primary consumers. (d) Change in food web topology following species loss and rewiring. Thick and thin lines denote strong and weak links, respectively. Red colour denotes lost species and links, green colour denotes rewiring consumers, their new resources and resulting new links, and grey nodes show already extinct species. Species are numbered (from left to right) as 1–6 (primary producers), 7–10 (primary consumers) and 11–12 (secondary consumers). Large arrows indicate at which point in time a species goes extinct. Small arrows identify consumer adjustments of feeding efforts (open) or rewiring (filled), where colour denotes the resource affected. No rewiring cost. Correlation in the response of species to environmental variation,ρ, equals 0.75. Figure 5: Network collapse driven by resource species extinctions and consumer rewiring. Time series showing population dynamics for ( a ) secondary consumers, ( b ) primary consumers and ( c ) primary producers. Horizontal dashed lines: extinction thresholds. Thick grey lines: combined densities of ( c ) all primary producers and ( b ) all primary consumers. ( d ) Change in food web topology following species loss and rewiring. Thick and thin lines denote strong and weak links, respectively. Red colour denotes lost species and links, green colour denotes rewiring consumers, their new resources and resulting new links, and grey nodes show already extinct species. Species are numbered (from left to right) as 1–6 (primary producers), 7–10 (primary consumers) and 11–12 (secondary consumers). Large arrows indicate at which point in time a species goes extinct. Small arrows identify consumer adjustments of feeding efforts (open) or rewiring (filled), where colour denotes the resource affected. No rewiring cost. Correlation in the response of species to environmental variation, ρ , equals 0.75. Full size image The scenario illustrated in Fig. 5 also suggests that the final community collapse can be quite abrupt and difficult to anticipate. Here the extinction of primary producer species decreases the intensity of interspecific competition among the producers, leading to strong density compensation at the producer level. This causes some consumer species to actually increase in abundance up to the point of network collapse. Monitoring of these populations would show positive trends over a large time span and hence suggest a low threat status while the opposite is actually the case—an extinction debt is present. We find that consumer rewiring is more likely to aggravate than to alleviate the effects of species loss—the risk of extinction cascades and system collapse increases. The explanation for this is that predator rewiring following prey species loss often leads to overexploitation of remaining prey species in the system, especially so if prey species cannot escape predation when rare and if predators are efficient in exploiting novel prey. Thus, even though rewiring can be advantageous for individual predators in the short term, it is likely to be harmful for long-term network persistence. Looking at the extinction patterns induced by rewiring (as illustrated by Fig. 5 ) from the point of view of trophic cascades, it is clear that both bottom-up and top-down processes are involved. This can be expected if the system in which a trophic cascade plays out consists of multiple and interconnected trophic chains. For example, in the simple case of two food chains emanating from the same basal species, a top-down effect along one chain will turn into a bottom-up effect along the other chain through the impact on the shared resource [6] , [33] . In the present study, the bottom-up effect of an initial resource extinction turns into a top-down effect, if consumers have the ability to switch to a new resource. We furthermore show that when this top-down effect is strong, that is, the added predation pressure is high, the new resource species may be driven extinct, at which point the cascade changes direction again. Indeed, the collapse illustrated in Fig. 5 takes place through a series of such directional changes in a strong ‘bouncing’ trophic cascade. A pre-requisite for this pattern to arise is the primary extinction of one or more resource species. Such extinctions should be expected to occur more frequently if the food web is subjected to an external stressor that more severely affects the resource species than it does their consumers. Nitrogen deposition, for example, is expected to cause extinctions at the primary producer level [34] . Because of their limited dispersal capacity plant species might also be more vulnerable to habitat fragmentation and global warming than many animal species [35] , [36] . Furthermore, increased natural environmental variation caused by climate change may also pose a greater risk to resources than to their consumers, at least in size-structured systems in which trophic level increases with body size. This is because a species’ life span tends to increase with average body size [37] and longevity can buffer the effects of environmental variation [38] . The strain from external stressors such as these may not only drive the primary extinctions, but could also increase the secondary extinction risk of resource species by making them more vulnerable to the increased predation pressure following a rewiring. Another condition for this pattern to arise is that the top-down effect from the rewiring consumer is strong enough to substantially reduce the abundance of the new resource. A dramatic example is provided by the sequential collapse of marine mammals in the North Pacific Ocean induced by prey switching (rewiring) killer whales. Following sharp declines in the great whales caused by large-scale commercial whaling, the killer whale switched to pinnipeds thereby decimating the populations of these species severely, which in turn lead to yet another prey switch to sea otters. The resulting decline in the sea otter populations finally led to local collapse of species-rich kelp forest ecosystems [24] , [25] . Another striking example involves large-scale rewiring in human exploitation of marine coastal fish and terrestrial mammals in West Africa [29] . Here years of poor fish supply—caused by previous intense fishing—coincided with increased hunting in nature reserves and sharp declines in abundances of several mammal species. There are several other examples showing that declining populations of preferred resource species lead to prey switching in consumers, although the consequences for the new prey species are less well-known, for example, ref. 39 . However, in some instances, concerns have been raised that such rewiring might lead to increased predation pressure on the new prey species with negative consequences for their persistence, for example, refs 40 , 41 . Under what circumstances is rewiring likely to cause substantial reductions in the abundance of the new prey species like in the examples above? Here we have shown that the risk of rewiring consumers overexploiting their new resource is smaller when (1) the consumers are less efficient in exploiting their new resource (high rewiring cost), (2) are less efficient at low resource densities (sigmoidal functional response), or (3) when food webs are dominated by generalist species. More generally, mechanisms that reduce the strength of trophic cascades would be expected to reduce the risk associated with consumer rewiring. In line with this expectation, we find that the factors identified above closely corresponds to, and supports, a set of hypotheses concerning trophic cascade strength [42] . The strength of top-down trophic cascades is hypothesized to decrease with decreased consumer efficiency, and accordingly we find weaker effects of rewiring consumers under such circumstances (1 and 2 above). Similarly, it has been suggested that the presence of prey refuges would decrease trophic cascade strength, by reducing the search efficiency of predators. The effect of the functional response (2 above) corresponds well also to this hypothesis, as one rationale for the sigmoidal functional response is the occurrence of a limited number of refuges. Weaker trophic cascades are also expected when interactions between trophic levels are weak or diffuse [42] . In line with this, we find the negative effect of rewiring on long-term network persistence to be weaker when consumers show equal preference for each of their prey species (generalist consumers), compared with when consumers show strong preference for one prey species (specialist consumers, 3 above). A generalist consumer losing one of its prey species will redistribute feeding efforts, and hence predation pressure, evenly among its remaining prey, imposing a weaker top-down effect compared with a specialist consumer losing its preferred prey. Moreover, in systems dominated by specialist consumers some prey species might be exposed to very high initial predation pressure, making them particularly vulnerable to an additional load caused by rewiring. In summary, the risk of extinction cascades is expected to be lower in networks with generalist consumers than in systems with specialist consumers. The impact of rewiring is also likely to depend on the strength of self-limitation (intraspecific competition). Specifically, top-down effects of rewiring is expected to be stronger if intraspecific competition in consumers is weak. Consumer densities will then be higher which will increase the risk of overexploitation of novel prey following rewiring and hence, the likelihood that prey density is supressed closer to the extinction threshold. This is in agreement with our analytical results for the simple 4-species community ( Fig. 4 ). The strength of interspecific competition among primary producers can also affect the impact of rewiring; if it is strong the positive effects of the loss of a competitor might counterbalance the negative effects of increased predation/grazing pressure caused by a new consumer and prevent the triggering of an extinction cascade ( Figs 4 and 5 ). We have here focused on the effects of extinction-induced rewiring in antagonistic networks like food webs. However, the consequences of rewiring could vary across network types. For instance, theoretical work suggests that extinction-induced rewiring in mutualistic networks like plant-pollinator systems is positive both at the species and the network level [19] (see also ref. 43 ). In a purely mutualistic system overexploitation is not an issue. However, a pollinating insect species can be engaged in both mutualistic and antagonistic interactions [44] having an herbivorous larvae stage that could potentially overexploit its host plants. The stability of networks containing a mixture of mutualistic and antagonistic interactions might differ from those that are purely antagonistic or mutualistic [45] , [46] . How extinction-induced rewiring would affect the persistence of stage-structured and other hybrid networks is an open and interesting question. Another interesting question is how rewiring might affect the topology of networks. For instance, interaction switches lead to increased nestedness in initially random mutualistic networks with potential consequences for their stability [47] , [48] . The effect of nestedness on the stability of mutualistic networks is a topic of considerable interest and debate (for example, refs 45 , 48 , 49 , 50 , 51 ). Another challenge is to disentangle how dispersal of individuals among local communities might affect the impact of rewiring. In open communities (metacommunities) spatial processes like re-colonization and rescue effects can potentially counterbalance local extinctions (for example, ref. 52 ) and hence rescue local food webs from extinction cascades. The potential for rescue effects to operate will depend on the rate of dispersal relative to the rate of extinction caused by increased predation pressure from rewiring consumers. Furthermore, it will depend on the spatial scale of movement of species at different trophic levels. Predators may often move over larger areas than their prey [53] and thus making it difficult for local prey populations to escape in space from high predation pressure. Also, mobile adaptive consumers can have a strong destabilizing effect on ecosystems if the spatial foraging scale of consumers is large compared with the spatial scale of the resource habitat [53] . Thus, spatial processes can have a destabilizing as well as a stabilising effect on ecological networks. Although many interesting questions remain to be explored, our study clearly reveals that adaptive rewiring may often aggravate rather than mitigate the consequences of species loss in antagonistic ecological networks like food webs. Indeed, rewiring constitutes an additional perturbation to the network since a rewiring consumer species in effect turns into a native invader [54] increasing the load on the remaining resource species. Thus, rewiring is a two-edged sword; it might be advantageous for individual consumer species in the short term, yet harmful for long-term network persistence. This finding has a bearing on the interaction of human harvesters with natural populations in that human harvesters are examples of especially flexible and efficient consumers [28] , [29] , [30] , [55] . Our study indicates that under such circumstances rewiring can potentially trigger extensive extinction cascades causing large changes in the structure and dynamics of ecosystems. Study systems Four natural food webs from different habitats are included in the analysis; Broadstone Stream [56] (running water), Kelp bed [57] (marine), Montane Forest [57] (terrestrial) and Phytotelmata [58] (freshwater) ( Fig. 3 , Supplementary Table 1 ). Nodes in the natural networks represent true species or trophic species, that is, functional or taxonomical groups that share resource and consumer nodes, and are here simply referred to as ‘species’. Species richness and connectance (proportion of possible trophic links that is realised—excluding any cannibalistic links) range from 17 to 28 and from 0.06 to 0.17, respectively ( Supplementary Table 1 ). For the food webs Broadstone Stream and Montane Forest the lowest trophic level are the primary consumers (herbivores) due to low resolution at the primary producer level. Each species on the lowest trophic level competes directly with all other species on that level and intraspecific competition is present in all species. Furthermore, we generate pyramidal model food webs with 12 and 24 species distributed over three trophic levels; primary producers, primary consumers and secondary consumers. The ratio between the numbers of species at the different trophic levels is 3:2:1. Trophic links are distributed randomly, but with some constraints: consumers must feed on at least one resource from the trophic level directly below themselves and cannibalism is not allowed. Secondary consumers can be omnivorous, that is, feeding not only on the primary consumers but also on the primary producers. Connectance is randomly drawn from the uniform interval [0.05 0.30]. Each primary producer species competes directly with all other primary producer species and intraspecific competition is present in all species. An additional set of model food webs are generated using the PNM [59] . The PNM uses a Gaussian formulation for the probability that species i eats species j . That is, there is always a non-zero probability that a species feeds on another species, and the closer the niche position of the resource is to the optimal diet position of the consumer, the higher the probability. This allows for gaps in the diet width of consumers. There are no constraints on trophic links except that cannibalism is not allowed. The size of the PNM food webs ranges between 12 and 21 species and connectance ranges between 0.02 and 0.35. Intra- and inter-specific competition is modelled as in pyramidal food webs. Finally, we generate a set of antagonistic bipartite model networks containing 12 basal and 12 herbivore species. We vary the degree of nestedness in these networks using the methods developed by Thébault and Fontaine [49] . Connectance, intra- and inter-specific competition is modelled as in pyramidal and PNM food webs. The analysed systems represent a broad spectrum of antagonistic network types and topologies; bipartite and pyramidal networks, networks generated by the probabilistic niche model algorithm and natural food webs from different habitats. Niche models like the PNM have been widely used to generate antagonistic networks. We also include pyramidal networks in our analysis since these networks have relatively discrete trophic levels, in agreement with the pattern found in real food webs [60] . Network dynamics Network dynamics are described by a generalized Rosenzweig–MacArthur model [22] , [61] : Here d N i /d t is the rate of change of the density of species i with respect to time in a network with S species, b i ( t ) is the per capita growth (mortality) rate for primary producers (consumers) of species i at time t and is the per capita effect of species j on the per capita growth (mortality) rate of species i . The interaction coefficients, , describes competitive and predator–prey (trophic) interactions. The functional response of predators to the densities of their prey is non-linear of type II (hyperbolic) or III (sigmoidal). Equation (1) can then be rewritten in a more detailed form as: Here competitive interactions are described by the first sum; a ij and a ii ( j=i ) is the per capita strength of inter- and intra-specific competition, respectively. The second and third sum describe the loss and gain of species i ’s density due to consumption. L ( i ) is the set of species being competitors to species i , C ( i ) is the set of species being consumers of resource species i , R ( j ) is the set of species being resources of consumer species j and R ( i ) is the set of species being resources of consumer species i . Further, h ij is the ‘preference’ (feeding effort) and α ij is the intrinsic attack rate of consumer species j on resource species i . T ij is the time needed for consumer i to catch and consume resource j (handling time), e ij is the rate at which resource j is converted into new consumer i (conversion efficiency) and q ij (capture exponent) is an interaction specific positive constant. The capture exponent ( q ) and handling time ( T ) determine the type of functional response: q =1 and T =0 gives a type I (linear) functional response; q =1 and T >0 gives a hyperbolic type II functional response and increasing q gradually from 1 to 2 gives an increasingly sigmoidal type III functional response. Environmental variability is introduced in species’ intrinsic growth or mortality rates as where is the mean per capita growth or mortality rate of species i and ɛ i ( t ) is a stochastic process defined by Here ɛ ik are independent and uniformly distributed stochastic values on the interval [−1 1], yielding a variance in ɛ of 0.333. Extreme values are as likely as the mean value of 0. The correlation among species in their response to environmental fluctuations ( ρ ), that is, the correlation between time series of ɛ ik is generated as in ref. 22 . We explore two scenarios: high ( ρ =0.75) and low ( ρ =0.25) correlation among species in their response to environmental variation. To get continuous time series of stochastic values, ɛ ik are then interpolated using a cubic spline interpolation method implemented in the Matlab function interp1. The resulting set of coupled ordinary differential equations are integrated over time using a variable order solver based on numerical differentiation formulas implemented in Matlab’s ode15s (model computer code available on request). We also indirectly account for demographic stochastic variation and other processes that affects small populations disproportionately by defining quasi-extinction thresholds (see Simulation). Adaptive rewiring and adjustment of feeding efforts It is plausible that extinction thresholds, set by processes like demographic stochasticity and Allee effects, could be higher than the density thresholds causing consumers to rewire. We therefore assume that rewiring and compensatory change in feeding efforts takes place in connection with the extinction of preferred prey species, and not before. Hence, an adaptive consumer adjusts its resource preferences (feeding efforts), h ij , when a resource in its original set of resources goes extinct. If the extinct resource was the preferred resource, another of its original resources is randomly chosen as preferred and h ij is updated for all its remaining resources so that h ij still sums to 1. If a non-preferred resource goes extinct, the remaining non-preferred resources will have their preferences increased while the preferred resource is unaffected. Finally, each time an adaptive consumer loses its last resource it rewires to a completely new resource from a trophic level below itself, thus forming a novel trophic link. Consumers with similar behavioural, physiological and morphological traits are likely to use similar types of resources. Thus, the new resource is randomly chosen from the set of resources belonging to the consumer which has the most similar set of prey as that of the rewiring consumer itself. Similarity of consumers with respect to their sets of prey species is quantified using the Jaccard index of similarity ( Fig. 1 ). We assume that rewiring entails a cost in the sense that the consumer is less effective in exploiting its new resource. Two cost scenarios are explored: a 75% (high cost) or a 25% (low cost) reduction of a consumer’s intrinsic attack rate, α ij , on the new resource species. Parameterization Mean intrinsic growth rates of primary producers, , are set to 1. Mean intrinsic mortality rates of consumers, , are randomly drawn from the uniform distribution [−0.01 −0.001] and ordered such that secondary consumers have lower intrinsic mortality rates than primary consumers (herbivores), that is, | b primary consumers |>| b secondary consumers |. This is because body mass of species often increases with trophic level [62] , [63] and larger body mass often confers lower mortality rates [64] . Direct interspecific competition among primary producers, a ij , is set to 0.5. There is no direct competition among consumer species—they only compete indirectly through shared resources. Intraspecific competition, a ii , is set to 1 for primary producers and to 0.01 for consumers. The intrinsic attack rate, α , and handling time, T , are assumed to be equal for all consumers and set to 1.5 and 0.2, respectively. The type of functional response is controlled by the capture coefficient q , which is set to 1 for a functional response of type II and 1.25 for type III. We vary the proportions of consumers with hyperbolic (type II) and sigmoidal (type III) functional responses as both types are likely to be present in a natural food web [65] and because the type of functional response of predators can have important consequences for the risk of extinction of their prey [66] . Conversion efficiency, e , is set to 0.2 for feeding interactions between adjacent trophic levels and to 0.02 for omnivorous links which are considered less efficient. Resource preferences (feeding efforts) of consumers, h ij , sum up to 1. Two scenarios with respect to prey preferences of consumers are analysed: (1) consumer species either show strong preference for one of their prey species (specialists) or (2) equal preference for each of their prey species (generalists). Specifically, in the specialist scenario consumers with more than one resource species show high preference ( h ij, high =0.9) for one of them (randomly assigned) while the preferences for the other resources are low and equal; h ij ,low =(1− h ij, high )/(no. of resources−1). In the generalist scenario consumers with more than one resource species show equal preference for each of them; h ij =1/(no. of resources). To verify the generality of our results we perform an expanded analysis covering a larger parameter space using LHS design [67] with randomised model parameters. This is done for a subset of the webs: 12-species pyramidal webs, PNM webs with 10 consumer species and the Phytotelmata food web. The selection of networks and scenarios used for this expanded analysis is based on representativeness and computational feasibility. Using LHS we first increase the parameter range analysed by setting the lower and upper interval limits of each of the 10 parameters to 0.5 and 2 times the constant parameter value used in the main analysis, respectively. Next, these larger intervals are divided into 10 equally sized sections (intervals). From each section a Latin Hypercube sample is randomly drawn to create a 10-dimensional Latin Hypercube that will hold 10 sets of parameter mean values, representing the larger parameter space ( Supplementary Table 3 ). Model parameter values are then randomly drawn from uniform intervals with the upper and lower interval limits set to the LHS parameter mean ±10%. The parameter sets that do not result in persistent networks (having species densities above predefined quasi-extinction thresholds) for at least 20,000 time units during a deterministic simulation, within 10,000 trials, are discarded. The remaining parameter sets are used in the analysis. We use the lhs-package (version 0.1) in R [68] to generate the Latin Hypercube. Simulation For the pyramidal model food webs, 12 and 24 species networks are simulated. Here, the number of consumer species is 6 and 12, respectively, (consumers constitutes 50% of the species in the webs). For the PNM food webs the number of consumers may not be equal in webs of the same size (total number of species). Here webs with 6 and 10 consumer species are simulated. The median number of species in these webs is 13 and 18 species, respectively. As in the pyramidal food webs, the consumers constitute 50% of all species in the bipartite model networks. Here networks with 24 species (that is, 12 consumer species) are simulated. The number of species in the 4 natural food webs are 17, 21, 27 and 28, respectively ( Supplementary Table 1 ). It was only possible (computationally feasible) to generate persistent (see below) models of the natural food webs for the strong prey preference (specialist) scenario. For all simulated network types and scenarios, the fraction of adaptive ( F Adap ) and non-adaptive (1- F Adap ) consumers as well as the fraction of consumer species having a functional response of type II ( F FR2 ) or type III (1- F FR2 ) is varied between 0 and 1 (in discrete steps corresponding to one consumer species). For each consumer trait combination within each scenario, 50 persistent replicates are generated. Networks are considered persistent if they remain feasible (having species densities above predefined quasi-extinction thresholds) for at least 20,000 time units during a deterministic simulation. As initial densities for this simulation we use the equilibrium densities from the corresponding system with a linear functional response (type I). These persistent networks are then integrated for another 10,000 time units (corresponding to ∼ 8000 generations for the primary producers and ∼ 30 generations for the longest lived consumer species in the theoretical webs), now with environmental stochasticity affecting intrinsic growth and mortality rates of species. As initial densities for these simulations we use the final densities from the deterministic simulation. Demographic stochasticity is implicitly modelled by defining quasi-extinction thresholds. The quasi-extinction thresholds are set to 0.002, 0.0002 and 0.00002 for primary producers, primary consumers and secondary consumers, respectively. However, the absolute levels are not of primary importance here since our aim is to compare relative extinction risks among the different scenarios explored, not to predict absolute extinction risks. If the density of a species falls below the quasi-extinction threshold it is considered extinct and is deleted from the system. A consumer species that has lost all prey species (and cannot rewire) will die from starvation. We assume that this starvation is not an instantaneous event, but a process that takes some time. During this time intermediate consumer can still interact with other species (that is, their predators), while top consumers cannot (at this point they will be isolated from all other species). Therefore intermediate consumers are kept in the system for 50 time steps following final prey loss, while top consumers are removed immediately. As a complement to the simulations we also study a simple 4-species system using analytical methods to get further insight of possible mechanisms involved. In this analysis, we also explore how the strength of interspecific competition among primary producers and the strength of intraspecific competition in consumers modulate the effects of rewiring. Statistical analysis To investigate potential influences of food web topology on the effect of rewiring on food web persistence a regression tree analysis [69] is performed. To this end, a set of network properties is calculated for each food web ( Supplementary Table 4 ). For each food web type, only properties that show variation among replicates are included in the analysis. Depending on food web type some of these properties show no variation among replicate webs, for example, the proportion of basal species is constant for all pyramidal food webs. In addition, nestedness is only included in the analysis of the bipartite webs, as calculating nestedness for networks with more than two trophic levels is far from trivial (but see ref. 70 ). The fraction of adaptive consumers ( F Adap ) and the fraction of consumers with a functional response of type II ( F FR2 ) are included in the analysis to better understand the relative importance of these predictors versus the food web topology. Consequently, the number of potential explanatory variables varies between the food web types (22 for PNM, 17 for pyramidal and 12 for bipartite food webs, Supplementary Table 4 ). All analyses described below are performed for each food web type independently. Inevitably, many network properties are related. To avoid an overly redundant set of explanatory variables we perform a correlation analysis. Network properties are removed so that no absolute value of pairwise correlation | ρ |>0.65 remains in the set. From clusters of network properties with high correlations between them, the most commonly used variable is used, for example, connectance among a larger group of link related properties. A screening analysis shows that our selection criteria of ‘convention’ did not result in the exclusion of any exceptionally powerful predictor (exceptional as compared with the power of the other properties within a certain correlation cluster). For the screening analysis we use generalized additive models (GAM) for estimating the explanatory power of each network property independently. A few exceptions to the cutoff rule of 0.65 are allowed in cases when two highly correlated properties are both deemed of great interest: for the bipartite food webs both nestedness (significant) and connectance ( ρ =0.88) are included and for the PNM webs both average trophic height and connectance ( ρ =0.75) are included in the regression analysis. However, by dropping either one of the properties from the set of explanatory variables and re-running the regression tree analysis with the diminished data set, we make certain that these exceptions do not negatively affect the performance of the analysis. After the selection process, the set of explanatory variables involved in the regression tree analysis consist of eight network properties for the PNM webs, seven properties for the pyramidal webs and five properties for the bipartite webs ( Supplementary Table 5 ). For each food web type four scenarios are analysed: specialist and generalist consumers; low and high rewiring cost ( Supplementary Figs 6–8 ). All analyses are performed in R (ref. 68 ; version 3.1.1 for correlation and screening analysis and 3.0.1 for the regression tree analysis). Package mgcv (version 1.7-23) is used for the GAMs of the screening analysis, using function gam with basis cr and basis dimension, k , set to 4 (see documentation for mgcv). Package mvpart (version 1.6-1) is used for the regression tree analysis, using function mvpart applying the 1SE rule, allowing a minimum of 10 data points in a leaf and running 1000 10-fold cross validations (see ref. 69 and documentation for mvpart). How to cite this article: Gilljam, D. et al. Adaptive rewiring aggravates the effects of species loss in ecosystems. Nat. Commun. 6:8412 doi: 10.1038/ncomms9412 (2015).